Codoping titanium dioxide nanowires with tungsten and carbon for enhanced photoelectrochemical performance Recent density-functional theory calculations suggest that codoping TiO 2 with donor–acceptor pairs is more effective than monodoping for improving photoelectrochemical water-splitting performance because codoping can reduce charge recombination, improve material quality, enhance light absorption and increase solubility limits of dopants. Here we report a novel ex-situ method to codope TiO 2 with tungsten and carbon (W, C) by sequentially annealing W-precursor-coated TiO 2 nanowires in flame and carbon monoxide gas. The unique advantages of flame annealing are that the high temperature (>1,000 °C) and fast heating rate of flame enable rapid diffusion of W into TiO 2 without damaging the nanowire morphology and crystallinity. This is the first experimental demonstration that codoped TiO 2 :(W, C) nanowires outperform monodoped TiO 2 :W and TiO 2 :C and double the saturation photocurrent of undoped TiO 2 for photoelectrochemical water splitting. Such significant performance enhancement originates from a greatly improved electrical conductivity and activity for oxygen-evolution reaction due to the synergistic effects of codoping. TiO 2 has been extensively investigated as a photoanode for photoelectrochemical (PEC) water splitting owing to its high photocatalytic activity, proper band-edge positions, superior photo-chemical stability, low-cost and non-toxicity [1] , [2] , [3] , [4] , [5] , [6] , [7] . Much research effort has been devoted to combat the large band gap of TiO 2 (~3.0–3.2 eV) [8] , [9] by using cationic [10] or anionic doping (or alloying, especially for high doping concentration) [11] , [12] , [13] . Although monodoping (single element doping) reduces the band gap of TiO 2 to some extent, it increases charge carrier recombination [10] , [14] and eventually decreases the overall PEC performance. Even without doping, the performance of TiO 2 -based PEC water-splitting cells is greatly limited by its rapid charge recombination due to the high trap densities in TiO 2 [4] . Recently, a new donor–acceptor codoping concept was proposed to improve the PEC water-splitting performance of TiO 2 photoanode because codoping TiO 2 with donor–acceptor pairs can reduce charged defects and their associated recombination, improve material quality, enhance light absorption and increase solubility limits of dopants [15] , [16] , [17] , [18] , [19] . According to density-functional theory calculations, various donor–accepter pairs, such as (W, C) [15] , [19] , (Mo, C) [15] , [16] , [19] , (2Nb, C) [15] , [18] , (2Ta, C) [15] , [18] , (W, 2N) [15] , [20] , (Ta, N) [15] , (Nb, N) [15] , (Sb, N) [21] , (Cr, N) [22] , (Zr, S) [15] and (Nb, P) [15] , have been proposed as good candidates for TiO 2 codoping on the basis of the modified band gaps and band-edge positions. Nevertheless, up to date, there is only indirect experimental evidence for the effects of codoping for PEC water splitting. For example, a number of metal/anion codoping pairs were shown to improve the photocatalytic activities of TiO 2 for organic pollutant decomposition due to enhanced visible-light absorption and charge separation [22] , [23] , [24] , [25] , [26] , [27] . Codoping ZnO with (Ga, N) led to highly conductive p-type ZnO film [28] , and improved PEC performance because of enhanced visible-light absorption and crystallinity [29] . Codoping LiFePO 4 with (Si, F) showed enhanced electrical conductivity and thus led to improved cathode rate performance for Li-ion batteries. [30] To our best knowledge, there is no direct experimental demonstration on the effect of codoping TiO 2 for PEC application because of the lack of suitable doping methods for donor (metallic) dopants. Previous methods of doping TiO 2 with metallic donors typically introduced the dopants during the synthesis stage of TiO 2 with methods, such as sol-gel [23] , [26] , [31] , hydrothermal [32] , sputtering [27] and solution combustion [33] . All these in-situ doping methods change the crystallinity/morphology compared with undoped TiO 2 , preventing the isolation of the doping effect from crystallinity/morphology effects on the PEC performance. Here we report a novel ex-situ sol-flame doping method to dope TiO 2 nanowires (NWs) with metallic dopants (donor), and C (acceptor) is subsequently doped into TiO 2 by conventional carbon monoxide (CO) annealing. The TiO 2 :(W, C) NWs double the saturation water oxidation photocurrent of undoped TiO 2 for PEC water splitting and outperform the monodoped samples (TiO 2 :W and TiO 2 :C). Moreover, such significant PEC enhancement is because the codoping TiO 2 with (W, C) significantly improves the electrical conductivity of TiO 2 and modestly enhances its activity for oxygen-evolution reaction (OER) as well. Ex-situ codoping of TiO 2 NWs The ex-situ codoping method for TiO 2 NWs is illustrated in Fig. 1 . First, rutile TiO 2 NWs with an average length of 2.8 μm and diameter of 100 nm are grown on fluorine-doped tin oxide (FTO) glass substrates by the hydrothermal method [34] , and the W-dopant precursor solution is prepared separately by the sol-gel method (see Methods section). Second, the TiO 2 NWs are dip-coated with the W-precursor solution (0.05 M) and then dried by air blowing, which leaves a uniform thin layer of W precursor on the surface of TiO 2 NWs. Next, the W-precursor-coated TiO 2 NWs are annealed in a 1,100 °C flame for 2 min that promotes the rapid diffusion of W into TiO 2 NWs. Finally, the W-doped TiO 2 NWs are annealed in gaseous CO at 550 °C for 30 min in a tube furnace. As such, TiO 2 NWs are successfully doped with the (W, C) donor–acceptor pair. 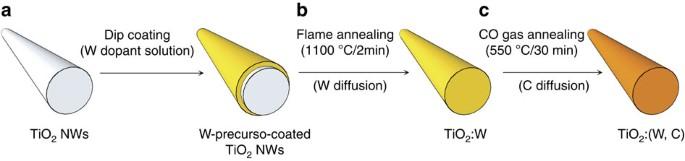Figure 1: Schematic illustration of theex-situdoping method. (a) The as-synthesized TiO2NWs grown by the hydrothermal method are dip-coated with W-precursor solution and then dried by air (or N2) blowing. (b) The W-precursor-coated NWs are annealed in a high-temperature flame (1,100 °C for 2 min) to enable rapid W diffusion. (c) The W-doped TiO2NWs are annealed in a tube furnace at 550 °C for 30 min under CO gas flow for C doping. Figure 1: Schematic illustration of the ex-situ doping method. ( a ) The as-synthesized TiO 2 NWs grown by the hydrothermal method are dip-coated with W-precursor solution and then dried by air (or N 2 ) blowing. ( b ) The W-precursor-coated NWs are annealed in a high-temperature flame (1,100 °C for 2 min) to enable rapid W diffusion. ( c ) The W-doped TiO 2 NWs are annealed in a tube furnace at 550 °C for 30 min under CO gas flow for C doping. Full size image Our ex-situ sequential doping method has several advantages. First, the most unique aspect of our doping method is the combination of sol-gel process and flame annealing (named as sol-flame) for doping W. Flame provides high temperature and an ultrafast heating rate to enable rapid dopant diffusion occurring in a very short time (a couple of minutes or less). Such brief high-temperature annealing minimizes morphology and crystallinity change of TiO 2 NWs. The flame-annealed TiO 2 :W NWs have almost identical morphology ( Supplementary Fig. S1a,b ) and crystallinity ( Supplementary Fig. S1e,f ) with that of as-synthesized (undoped) TiO 2 NWs. When the W-precursor-coated TiO 2 NWs are annealed in a conventional furnace, the slow heating rate of the furnace limits the annealing temperature to be not more than 600 °C to protect the FTO substrates. As a result, WO 3− x particles are formed on the surface of TiO 2 NWs instead of diffusing into TiO 2 ( Supplementary Fig. S1c ). Furthermore, even with rapid thermal annealing at 1,100 °C using the furnace (that is, preheating the furnace to 1,100 °C first and then quickly inserting the sample), cracks are generated in glass substrate due to thermal stress ( Supplementary Fig. S1d ), showing the advantage of flame annealing. Second, the ex-situ doping approach, that is, incorporating dopants after NW growth, can be broadly applied to various metal-oxide NWs regardless of their synthesis methods. Third, the sequential doping process enables independent control and optimization of doping conditions for each dopant ( Supplementary Fig. S2 ). It should be noted that our doping methods are applicable to other donor–accepter pairs as well. We have tested other codoping pairs, including (Nb, C) and (Ta, C), and they also exhibit better PEC performance than the Nb, Ta or C monodoped TiO 2 and undoped TiO 2 ( Supplementary Fig. S3 ). Morphology and dopants distribution The morphology and dopant profiles of TiO 2 :(W, C) NWs are illustrated in Fig. 2 . The cross-sectional and top views ( Fig. 2a ) show that the TiO 2 :(W, C) NWs have an average diameter of 100±10 nm, length of 2.8±0.1 μm and surface coverage density around 6.3 × 10 9 NWs per cm 2 . The energy-dispersive X-ray spectrometer mapping, together with transmission electron microscope (TEM) image, ( Fig. 2b ), clearly shows that both W and C are doped over the entire TiO 2 NW. The surface concentrations of W and C dopants are estimated to be ~10.2±2.0 at.% and 13.1±3.0 at.%, respectively, via a quantitative analysis of the low loss and core-loss electron energy loss spectroscopy (EELS) spectra ( Supplementary Fig. S4 ). The W and C dopant radial depth profiles within TiO 2 NWs are analysed by the secondary ion mass spectrometry (SIMS) measurements for which we use larger TiO 2 :(W, C) NWs with an average diameter of ~300 nm for higher secondary ion yield (Methods section and Supplementary Fig. S5 ). 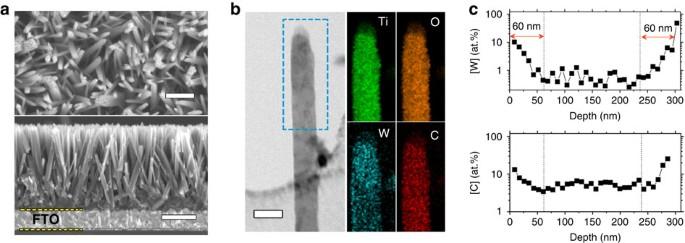Figure 2: Morphology and dopant-distribution characterization. (a) Top-view and cross-sectional scanning electron microscopy images. Scale bar, 500 nm (top view) and 1 um (cross-sectional). (b) TEM and energy-dispersive X-ray spectrometer mapping images. Scale bar, 100 nm. (c) SIMS analysis of radial depth profiles for W and C. Figure 2c shows the radial depth profiles of W and C dopants, which are normalized by Ti and O counts, respectively. For both W and C, their depth profiles show that the dopant concentration is high near the surface and then decreases along the radial direction towards the centre. The relatively symmetric shape of W and C dopant profiles along the diameter of the NW indicates homogeneous radial diffusion of W and C. The SIMS profiles show that the radial diffusion depths for both W and C are about 60 nm, so our TiO 2 NWs (~100 nm diameter) used for PEC tests are fully doped with W and C dopants, which is confirmed by EELS analysis ( Supplementary Fig. S4 ). Figure 2: Morphology and dopant-distribution characterization. ( a ) Top-view and cross-sectional scanning electron microscopy images. Scale bar, 500 nm (top view) and 1 um (cross-sectional). ( b ) TEM and energy-dispersive X-ray spectrometer mapping images. Scale bar, 100 nm. ( c ) SIMS analysis of radial depth profiles for W and C. Full size image PEC water-splitting performance The PEC water-splitting performance of the codoped TiO 2 :(W, C) NWs is evaluated by measuring photocurrent density–potential ( J–V ) curves using a standard three-electrode configuration under air mass (AM) 1.5 G simulated solar light illumination (100 mW cm −2 ), and compared with undoped and monodoped (W and C) TiO 2 NWs ( Fig. 3a ). The monodoped TiO 2 NWs are prepared by using the identical doping conditions as the TiO 2 :(W, C) samples. First, the photocurrent density of the undoped TiO 2 NWs is 0.75 mA cm −2 at 1.23 V RHE , which is comparable to previously reported values. [34] , [35] Second, both monodoped TiO 2 :W and TiO 2 :C NWs, in comparison with the undoped TiO 2 NWs, show much higher photocurrent density values, that is, 1.22 and 1.41 mA cm −2 , respectively, at 1.23 V RHE . More importantly, the codoped TiO 2 :(W, C) NWs have the highest photocurrent density of 1.81 mA cm −2 at 1.23 V RHE , which is about 2.4 times higher than that of undoped TiO 2 NWs, supporting the effectiveness of using donor–acceptor pairs to enhance PEC performance as suggested by previous theoretical calculations [15] , [19] . To the best of our knowledge, this is the first experimental demonstration for a donor–acceptor codoped TiO 2 system that exhibits enhanced PEC water-splitting performance than monodoped TiO 2 . Finally, the stability of the codoped TiO 2 :(W, C) NWs is evaluated by measuring the photocurrent–time ( J–t ) response ( Fig. 3b ). In the given 30-min experimental time interval, no obvious degradation of the photocurrent is observed. Significantly, even after over 6 months of storage in a strong base (2 M KOH) solution, the J–V curve of the codoped TiO 2 :(W, C) NWs remains unchanged ( Supplementary Fig. S6 ), indicating the excellent chemical stability of the TiO 2 :(W, C) NWs. 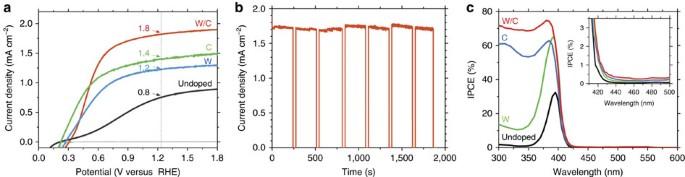Figure 3: Comparison of PEC performance. (a) Photocurrent-potential (J–V) curves of undoped, W-doped, C-doped and (W, C)-codoped TiO2NWs measured in a three-electrode setup (TiO2working, Pt-wire counter, SCE reference electrode, scan rate of 50 mV s−1) and 1 M KOH electrolyte under simulated solar light illumination (AM 1.5 G, 100 mW cm−2). (b) The photocurrent density-time response shows good stability of TiO2:(W, C). (c) IPCE spectra measured at 1.23 V versus RHE. The inset shows a magnified view in the wavelength region of 400–500 nm. Figure 3: Comparison of PEC performance. ( a ) Photocurrent-potential ( J–V ) curves of undoped, W-doped, C-doped and (W, C)-codoped TiO 2 NWs measured in a three-electrode setup (TiO 2 working, Pt-wire counter, SCE reference electrode, scan rate of 50 mV s −1 ) and 1 M KOH electrolyte under simulated solar light illumination (AM 1.5 G, 100 mW cm −2 ). ( b ) The photocurrent density-time response shows good stability of TiO 2 :(W, C). ( c ) IPCE spectra measured at 1.23 V versus RHE. The inset shows a magnified view in the wavelength region of 400–500 nm. Full size image The incident photon-to-current conversion efficiencies (IPCEs), equivalent to external quantum efficiency, of four samples (undoped, W-doped, C-doped and W/C-codoped TiO 2 NWs) are measured at 1.23 V RHE where the photocurrent density values for all the samples are saturated. The IPCE values are plotted versus wavelength in Fig. 3c to compare the wavelength-dependent photocurrent response for the four TiO 2 NWs. First, the codoped TiO 2 :(W, C) NWs have the highest IPCE values (IPCE max ~80% at 380 nm) throughout the whole wavelength region below the band gap (~420 nm), and then the IPCE values are lowered in the order of C-doped (IPCE max ~66% at 385 nm), W-doped (IPCE max ~64% at 390 nm) and undoped TiO 2 (IPCE max ~32% at 395 nm). Second, the codoped TiO 2 :(W, C) NWs shows noticeable though very weak IPCE response at the visible-light region (>420 nm). IPCE of a PEC photoelectrode is determined by the efficiencies of three fundamental processes involved in PEC water-splitting reaction as illustrated in equation (1), that is, charge generation efficiency ( ), charge transport efficiency within the material ( η transport ) and charge transfer (collection) efficiency at the electrode/electrolyte interface ( η transfer ). [8] To identify the key factors responsible for the high IPCE for the TiO 2 :(W, C) NWs, the individual contributions of the above three factors are investigated separately. First, the light-absorption properties of the four TiO 2 samples (undoped, W-doped, C-doped and W/C-codoped) are measured (see Methods section) and compared over a wavelength range from 300 to 650 nm ( Fig. 4a ). 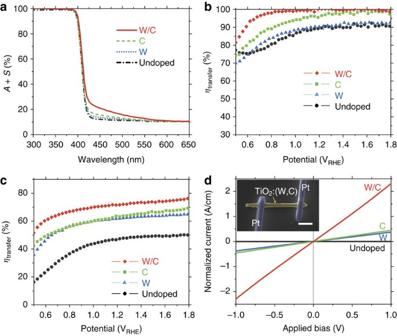Figure 4: Comparison of optical, charge transport and charge transfer properties. (a) Light absorption (plus scattering) of undoped (black), W-doped (blue), C-doped (green) and (W, C)-codoped TiO2NW (red) arrays grown on quartz. The integrated light absorption (plus scattering) values calculated by integrating over the wavelength, are 59.5%, 60.7%, 61.1% and 64.0% for undoped, W-doped, C-doped, and (W, C)-codoped TiO2NWs, respectively. (b) Charge transport efficiencies. (c) Charge transfer efficiencies. (d) Current–voltage curves of single NW. The inset shows the scanning electron microscopy image of single TiO2:(W, C) NW with metal (Pt) contacts at both ends. Scale bar, 1 μm. Figure 4a shows the light-absorption spectra of the four TiO 2 NW arrays grown on quartz substrates. Although the TiO 2 :(W, C) NWs show slightly higher visible-light absorption tails in the wavelength region of 420–580 nm, its integrated light absorption (~64%) over 300–580 nm is comparable to the other three samples, indicating that codoping within our doping conditions has little impact on the light absorption or charge generation efficiency ( ). Figure 4: Comparison of optical, charge transport and charge transfer properties. ( a ) Light absorption (plus scattering) of undoped (black), W-doped (blue), C-doped (green) and (W, C)-codoped TiO 2 NW (red) arrays grown on quartz. The integrated light absorption (plus scattering) values calculated by integrating over the wavelength, are 59.5%, 60.7%, 61.1% and 64.0% for undoped, W-doped, C-doped, and (W, C)-codoped TiO 2 NWs, respectively. ( b ) Charge transport efficiencies. ( c ) Charge transfer efficiencies. ( d ) Current–voltage curves of single NW. The inset shows the scanning electron microscopy image of single TiO 2 :(W, C) NW with metal (Pt) contacts at both ends. Scale bar, 1 μm. Full size image Furthermore, the charge transport efficiency ( η transport ) and charge transfer efficiency ( η transfer ) are decoupled and quantified by using H 2 O 2 as a hole scavenger approach (see Methods section) [36] . The estimated charge transfer and transport efficiencies of the four TiO 2 samples are compared in Fig. 4b . For the estimated charge transfer efficiency ( Fig. 4b ), because the rutile TiO 2 , especially the (110) terminated surface, has high catalytic activity towards OER, [37] , [38] , all of the four TiO 2 samples show relatively high charge transfer efficiencies exceeding 70% throughout the whole potential range. Furthermore, the codoped TiO 2 :(W, C) NWs sample has the highest charge transfer efficiency (99%) at 1.23 V RHE , in comparison with the undoped (89%), W-doped (91%) and C-doped (96%) samples. The observed charge transfer efficiency difference suggests that the presence of donor–acceptor pair effectively reduces the surface recombination of charge carriers, especially at the low potential region (<1.0 V RHE ). The OER activity is also improved on monodoped rutile TiO 2 (110) surface that is consistent with the recent theoretical predication based on density-functional theory calculations. [39] Previous experimental studies also suggest that the monodoping can induce high surface acidity and increase of reactant adsorption, [40] , [41] enhancing the charge transfer process. Finally, though the codoped TiO 2 :(W, C) NWs improves the charge transfer efficiency approximately by 10%, the improvement is not large enough to explain its 2.4 times higher saturation photocurrent density value. The third and last factor affecting the IPCE value is the charge transport efficiency, for which both electron and hole transport is important and mostly affected by the bulk recombination process. As shown in Fig. 4c , the codoped TiO 2 :(W, C) NWs sample has the highest estimated charge transport efficiency (50–80%), on average over two times higher than that of the undoped TiO 2 NWs. The transport efficiency for monodoped TiO 2 :W and TiO 2 :C samples are in between those of the codoped and undoped samples, very similar to the PEC performance shown in Fig. 3a . The electron-transport property is further compared by measuring the conductivity of individual TiO 2 NWs (see Methods section). Figure 4d shows linear current–voltage ( I–V ) curves for four individual TiO 2 NWs, indicating good ohmic contact. The calculated electrical conductivity values of the undoped, W-doped, C-doped and W/C-codoped samples are ~0.0001, 0.37, 0.46 and 2.26 S cm −1 , respectively. The W-doped, C-doped and W/C-codoped samples have over three orders of magnitude higher conductivity than the undoped sample, suggesting that doping TiO 2 with W and/or C significantly improves the electron-transport property. It should be noted that codoping gives higher conductivity improvement than the monodoping cases, indicating the defect passivation effect by codoping of W (donor) and C (acceptor). On the other hand, the improvement of charge transport efficiency is much lower than the increase of the electrical conductivity, suggesting that the bulk recombination, likely hole transport, is still the bottleneck for the overall charge transport process. Considering all the three factors, that is, light absorption, charge transport and transfer properties, the most pronounced effect of codoping for TiO 2 is to improve the charge transport property, that is, increasing electrical conductivity, and a minor effect is to improve the surface OER activity. We further synthesized W/C-codoped TiO 2 NWs with higher doping concentration (W/C no. 2) than the optimally codoped TiO 2 : (W, C) NWs (W/C no. 1, the sample discussed above) by using higher molar concentration of W-precursor solution (0.1 M) and longer duration of CO gas annealing (550 °C for 1 h). As shown in Fig. 5a–c , the W/C no. 2 has much higher W (17.5 at.%) and C (18.3 at.%) surface doping concentrations than the W/C no. 1 (optimal sample for PEC, W: 10.2 at.%, C: 13.1 at.% at the NW surface). Even though the W/C no. 2 has such high W- and C-doping concentrations, there is no nanoparticle formation at the TiO 2 NW surface and the high-resolution TEM images at the region of A, B and C ( Fig. 5a ) also confirms that the W/C no. 2 remains to be highly crystalline without dopant segregation. In comparison with the W/C no. 1, the W/C no. 2 exhibits inferior PEC water-splitting performance with lower saturation photocurrent density and lower IPCE values (especially near the band-edge wavelength region, 360–400 nm) ( Fig. 5d ). Finally, both W/C no. 1 and W/C no. 2 exhibit <1% IPCE values in the visible-light wavelength region (420–550 nm). To identify the reasons for the lower performance of W/C no. 2, we again determine the individual efficiency of the three processes that governs the PEC water-splitting performance, that is, light absorption (charge generation), charge transport and charge transfer efficiency, as shown in Fig. 5f–h . First, the visible-light absorption (>420 nm) of the W/C no. 2 with higher W- and C-doping concentrations is obviously higher than that of the W/C no. 1 sample ( Fig. 5f ). Nevertheless, the IPCE in this visible-light region is nearly zero. Second, the charge transfer efficiency of W/C no. 2 is lower than that of W/C no. 1, especially at lower applied potential region ( Fig. 5g ). It is likely due to decreased OER activity by higher W and C concentration at the TiO 2 surface [10] . Third, the charge transport efficiency of W/C no. 2 is consistently lower than that of W/C no. 1 over the entire applied potential range ( Fig. 5h ). This large decrease of charge transport efficiency in W/C no. 2 likely comes from the decreased conductivity due to the enhanced dopant scattering effect at much higher doping concentration. [42] As a result, though the TiO 2 NWs with higher doping concentration of W and C dopants exhibit increased visible-light absorption, their IPCE in the visible light range is still very weak (about 0.5%). In addition, the TiO 2 NWs with higher doping concentration of W and C dopants exhibit lower charge transport and charge transfer efficiencies, and hence lower PEC performance than those of the optimal sample. 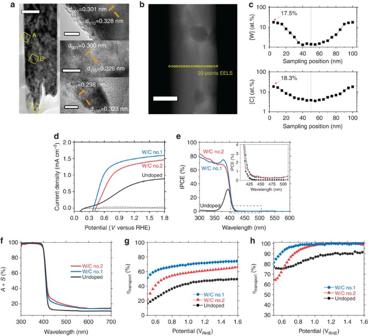Figure 5: Characterization and PEC water-splitting performance of TiO2NWs with high W- and C-doping concentrations. (a) TEM and high-resolution TEM images of W/C no. 2 (W: 17.5 at.%, C: 18.3 at.% at the NW surface). Scale bar, 50 nm (TEM) and 5 nm (high-resolution TEM). (b) STEM image. Scale bar, 50 nm. (c) Concentration profiles of W and C dopants along the NW diameter in W/C no. 2. Comparison of W/C no. 1 (blue) and W/C no. 2 (red) with (d), three electrodesJ–Vcurves (W/C no. 1, W: 10.2 at.%, C: 13.1 at.% at the NW surface), (e) IPCE, (f) light absorption (quartz substrate), (g) charge transfer efficiency and (h) charge transport efficiency. The data of undoped TiO2NWs (black) are added for reference. Figure 5: Characterization and PEC water-splitting performance of TiO 2 NWs with high W- and C-doping concentrations. ( a ) TEM and high-resolution TEM images of W/C no. 2 (W: 17.5 at.%, C: 18.3 at.% at the NW surface). Scale bar, 50 nm (TEM) and 5 nm (high-resolution TEM). ( b ) STEM image. Scale bar, 50 nm. ( c ) Concentration profiles of W and C dopants along the NW diameter in W/C no. 2. Comparison of W/C no. 1 (blue) and W/C no. 2 (red) with ( d ), three electrodes J–V curves (W/C no. 1, W: 10.2 at.%, C: 13.1 at.% at the NW surface), ( e ) IPCE, ( f ) light absorption (quartz substrate), ( g ) charge transfer efficiency and ( h ) charge transport efficiency. The data of undoped TiO 2 NWs (black) are added for reference. Full size image In summary, we report the first experimental demonstration that codoping TiO 2 NWs with W and C indeed greatly enhances the PEC water-splitting performance compared to the monodoped and undoped TiO 2 NWs. Our novel ex-situ sol-flame doping method effectively dopes TiO 2 NWs with W without changing the morphology and crystallinity of TiO 2 NWs and without damaging the delicate FTO substrate. The codoped TiO 2 :(W, C) NWs exhibit improved saturation photocurrent density than monodoped TiO 2 :W and TiO 2 :C and 2.4 times higher saturation photocurrent density than the undoped TiO 2 NWs, and the enhancement is attributed to mainly charge transport efficiency improvement and minor charge transfer efficiency improvement. We believe that the effectiveness of our doping method and codoping strategies, together with theoretical guidance, will enable further improvement of the PEC water-splitting performance of many other metal-oxide photoanodes. Synthesis of rutile TiO 2 NWs array The pristine TiO 2 NW arrays were synthesized on TiO 2 nanoparticle-coated FTO substrates using the hydrothermal method, and the details were reported in our previous work [34] . Briefly, for a typical synthesis, 0.6 ml of titanium (IV) butoxide (Aldrich Chemicals, 97%) was added into 50 ml of an aqueous HCl solution (25 ml of deionized (DI) water+25 ml of concentrated HCl (38%)) under magnetic stirring. For the growth of larger diameter TiO 2 NWs that were used for the SIMS analysis, larger amount of Ti-butoxide (1 ml) was added and the growth substrate was quartz. After stirring for another 5 min, the solution was poured into a Teflon-lined stainless steel autoclave (100 ml capacity), and pieces of the TiO 2 nanoparticle-coated FTO substrates, which have been cleaned for 10 min using an ultrasonicator in a mixed solution of DI water, acetone and isopropanol (IPA), were immersed in the solution. The autoclave was sealed and heated to 170 °C in an oven, and held at 170 °C for 7 h. The autoclave was then removed from the oven and allowed to cool to room temperature naturally on the bench top. The obtained products were washed with DI water and finally annealed at 450 °C for 1 h in air. Preparation of W-dopant precursor solution The W-dopant precursor solutions with metal salt concentrations of 0.01–0.2 M were prepared by using tungstic acid (H 2 WO 4 , 99%; Sigma-Aldrich Chemicals), hydrogen peroxide (H 2 O 2 , 30%; Sigma-Aldrich Chemicals) and 2-methoxyethanol (C 3 H 8 O 2 , >99%; Acros Organics) with a three-step sol-gel method: (1) dissolving the desired amount of H 2 WO 4 into 6–10 ml of H 2 O 2 , (2) removing excess H 2 O 2 and water by evaporation of the solution on a hot plate (130 °C) until the amount of the remained solution was about 1 ml and (3) mixing the 1 ml solution with 2-methoxyethanol by sonication (5 min) and stirring (1 h). After aging for 6–12 h, the prepared precursor solution was used for dip-coating the as-synthesized TiO 2 NWs. Doping TiO 2 NWs with W and/or C (i) To dope W into TiO 2 NWs, the prepared W-precursor solution was coated over the entire surface of TiO 2 NWs by the dip-coating method [43] , [44] . After drying by air (or N 2 ) blowing and subsequent air-annealing at 80 °C for 10 min, the W-precursor-coated TiO 2 NWs were annealed in a premixed flame of 1,100 °C for 2 min with a stoichiometric fuel-to-oxidizer equivalence ratio (Φ) of 1.0 (the flow rates of CH 4 and air were 2.0 and 25.5 SLPM (standard liters per minute), respectively). [43] , [44] The stoichiometric condition and usage of CH 4 minimizes the possibility of forming oxygen vacancy and carbon deposition on the TiO 2 NWs. (ii) For the C doping, the as-synthesized or W-doped TiO 2 NWs were annealed in a tube furnace (550 °C for 30 min) with 30 sccm CO gas flow. For codoping of W and C, sequential doping process of (i) and (ii) was used. The dependence of PEC performance on the doping conditions is discussed in detail in Supplementary Fig. S2 . Material characterizations and dopant depth profiles The morphologies of undoped and doped TiO 2 NWs were investigated using a scanning electron microscopy (FEI XL30; Sirion). The dopant distribution and surface concentration were investigated using a TEM (F20 FEI Tecnai, 200 kV) equipped with an energy-dispersive X-ray spectrometer and an EELS ( Supplementary Fig. S4 ). SIMS measurements were conducted to analyse the radial depth profiles of W and C in TiO 2 :(W, C) NWs. To increase the secondary ion yield for SIMS measurement, larger diameter TiO 2 NWs (~300 nm) were grown on quartz substrates using larger amount of Ti-butoxide (1 ml) addition. After doping with W and C, the TiO 2 :(W, C) NWs were sonicated in IPA. The NW suspension was then drop-cast onto a piece of Si (100) wafer to disperse TiO 2 NWs on the Si substrate. To remove the solvent residue, the NW-deposited Si substrate was washed with DI water and dried in a vacuum. The SIMS measurements were carried out using a Cameca NanoSIMS-50. A Cs + primary ion beam, accelerated at 16 keV with a 3.6 pA beam current, was used to sputter the surface of the NWs. The 12 C, 18 O, 28 Si, 48 Ti, 48 Ti 16 O and 184 W 16 O secondary ions and ionic fragments were collected and analysed in a mass spectrometer. The rastered area was 1 × 1 μm 2 and the gated/analysis area was the centre 0.25 μm 2 area to ensure that the collected counts only come from the NWs ( Supplementary Fig. S5 ). The sputtering rate was estimated by using the TiO 2 NW diameter and the depth profile of 28 Si. Optical measurements As FTO and the underlying glass can contribute to background absorption in the longer wavelength regime, TiO 2 NWs for the optical measurements were grown on the quartz substrate instead. The wavelength-dependent optical absorption properties were obtained with an integrating sphere using a xenon lamp coupled to a monochromator (Model QEX7; PV Measurements, Inc.). The absorption plus scattering was calculated from these measurements with the formula A + S =1−T−R, where A is the absorption, S is the scattered light that was not accounted for in the measurement, T is the total transmittance and R is the total reflectance. Electronic transport properties measurement To measure electronic transport properties of single TiO 2 NWs, the NWs were sonicated in IPA and then drop-cast onto a SiO 2 /Si substrate [45] . Platinum (Pt) metal contacts were deposited on the both ends of each TiO 2 NWs by using the focused ion beam (FEI Strata DB235) [46] . Current–voltage ( I–V ) measurements were conducted at room temperature using a semiconductor analyser (Model 4200-SCS; Keithley) with tungsten probes. PEC measurements The PEC performance of undoped and doped TiO 2 NWs was measured using a potentiostat (Model SP-200; BioLogic) in a three-electrode configuration (a saturated calomel reference electrode (SCE) and a Pt-wire counter electrode) under illumination of simulated solar light (AM 1.5 G, 100 mW cm −2 ) using solar simulator (Model 94306A, Class AAA; Oriel). Before the measurement, the solar simulator intensity was calibrated with a reference silicon solar cell and a readout metre for solar simulator irradiance (Mode 91150V; Newport). The illuminated area of the working TiO 2 electrode was 0.63 cm 2 defined by a mask. A volume of 1 M KOH or 1 M KOH with 0.5 M H 2 O 2 solution was used as the electrolyte. During the PEC measurement, the electrolyte was deaerated by Ar purging to remove the dissolved oxygen. In a typical J–V measurement, the voltage was swept linearly from −1.0 to 2.0 V SCE at a scan rate of 50 mV s −1 . The IPCE was measured at 1.23 V RHE (=~0.2 V SCE ) using a specially designed IPCE system for solar cell (QEX7; PV measurements), with three-electrode configuration. A 75-W Xe lamp equipped with a monochromator (CM-110, 1/8; SP Spectra Product) was used to generate a monochromatic beam. The incident light intensity was calibrated by a standard silicon photodiode. The charge transport and transfer efficiencies were estimated as functions of applied potential by using H 2 O 2 as a hole scavenger under AM 1.5 G simulated solar light illumination [36] . The key assumption for this approach is that the oxidation kinetics of H 2 O 2 is very fast and its charge transfer efficiency is 100%, so the ratio of photocurrent density measured in H 2 O and H 2 O 2 gives the charge transfer efficiency ( η transfer ) for H 2 O (equation 2). The charge transport efficiency ( η transport ) was further calculated by dividing photocurrent density in H 2 O 2 by the total light-absorption efficiency ( ), which is obtained from integration of light absorption ( Fig. 4a ) with respect to the AM 1.5 G solar light spectrum (equation 3). How to cite this article: Cho, I. S. et al . Codoping titanium dioxide nanowires with tungsten and carbon for enhanced photoelectrochemical performance. Nat. Commun. 4:1723 doi: 10.1038/ncomms2729 (2013).